The fitness of dispersing spotted hyaena sons is influenced by maternal social status Life history theory predicts that mothers should provide their offspring with a privileged upbringing if this enhances their offspring's and their own fitness. In many mammals, high-ranking mothers provide their offspring with a privileged upbringing. Whether dispersing sons gain fitness benefits during adulthood from such privileges (a 'silver spoon' effect) has rarely been examined. In this paper, we show that in the complex, female-dominated society of spotted hyaenas, high-born sons grew at higher rates, were more likely to disperse to clans offering the best fitness prospects, started reproducing earlier and had a higher reproductive value than did lower-born sons. This illustrates the evolutionary importance of maternal effects even in societies in which male size or fighting ability does not influence fitness. By demonstrating for the first time in a non-human mammal that maternal status influences immigration patterns, the study also advances our understanding of two key ecological and evolutionary processes, dispersal and habitat selection. The environment that an offspring experiences during development can have pronounced consequences on its growth, behaviour, survival and reproductive success [1] , [2] , [3] , [4] , [5] . In many species, the most significant environment that offspring experience during their development is the maternal environment [6] , [7] . According to life history theory, mothers should invest in their offspring if this enhances offspring survival and fitness, and if the fitness benefit to mothers from increased offspring fitness exceeds the cost of their investment [8] . Whether the maternal environment influences the fitness and reproductive value of sons is unknown in most mammals because male mammals usually disperse and, thus, few studies have matched maternal quality to the fitness and reproductive value of sons after dispersal. In the red deer ( Cervus elaphus ), a species with pronounced sexual dimorphism, in which male fitness is linked to body size and fighting ability, a privileged upbringing by a mother of high social status provides sons with fitness benefits during adulthood [9] . Whether a privileged upbringing also provides fitness benefits to sons in multifemale multimale mammal societies in which male fitness depends on how well males conform to female mate-choice preferences rather than a male's fighting ability or body size is currently unknown [10] . Previous empirical studies on social mammals with high maternal investment documented that the maternal environment influences the quality and fitness of daughters [11] , [12] , [13] , [14] , [15] . In these societies, females usually remain in the group in which they were born, form matrilines with related females and create linear dominance hierarchies [16] , [17] . Because socially dominant females have preferential access to environmental resources, there is usually a strong positive relationship between female social status and female reproductive success [14] , [18] , [19] . In many of these species, daughters acquire a dominance position close to and below that of their mother [11] , [12] , [13] , [15] . As a result, daughters of high-ranking females grow faster, survive better and enjoy the fitness benefits associated with a high social status [14] , that is, they benefit from a 'silver spoon' effect [20] . In the spotted hyaena ( Crocuta crocuta ) ( Fig. 1 ), a large carnivore with minimal sexual dimorphism [21] , [22] that lives in highly structured, female-dominated social groups termed clans [23] , access to resources is strictly status related [16] , and females of high social status have a higher reproductive value and success than do females of low social status [14] . Post-natal maternal investment is exceptionally high, involving the production of milk of high nutrient content [24] during a long lactation period of up to 2 years (this study). Offspring of both sexes acquire a social position immediately below that of their mother during adolescence through a behavioural mechanism in which mothers support their offspring during interactions with clan members that they dominate [13] , [14] , [15] . A study of adopted offspring reared by surrogate mothers found no evidence of a direct maternal genetic effect, or a maternal androgen effect during gestation, on the rank that adopted offspring obtained at adulthood [15] . Female offspring usually remain in their natal clan [25] and retain their social status during adult life, provided they retain behavioural support of a close female relative [14] , [26] . Offspring of high-ranking females grow faster and their daughters start reproducing at a younger age and have higher reproductive success than do daughters of low-ranking females [14] . In contrast, male offspring usually leave the natal clan and immigrate into another clan [27] . They join the new clan at the bottom of the male social hierarchy, observe strict conventions of social queuing and increase in status with increasing tenure when higher-ranking males emigrate or die [28] . 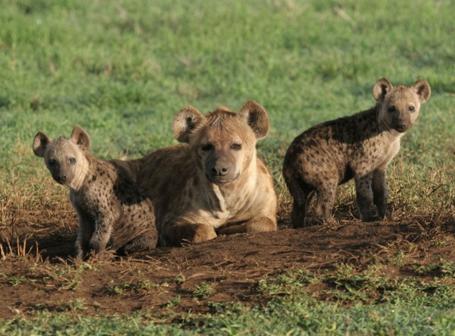Figure 1 Spotted hyaena mother with her two 3.9-month-old cubs. Figure 1 Spotted hyaena mother with her two 3.9-month-old cubs. Full size image Male reproductive success in spotted hyaenas strongly depends on how well males conform to female mate-choice preferences [27] , [29] because females exercise considerable mate choice [29] and have complete control over mating, owing to the unusual anatomy of their outer reproductive organs [26] . Successful males are those that join clans with high numbers of females likely to choose them as sires [27] , and males that build long-term, friendly relationships with females [29] . In contrast to some other social mammals [30] , [31] , [32] , the reproductive success of male spotted hyaenas is not directly related to their social status and there is no evidence that body size or fighting ability influences male fitness [29] , [33] . In such a system, the quality of a mother may influence the performance of her sons in a number of indirect ways. Better growth during the nursing period and preferential access to food until dispersal might increase the likelihood of sons of high-quality females to survive to immigration [34] , [35] , enable them to start producing offspring at a younger age [36] and attain a longer adult lifespan or tenure in a group [37] than sons of low-quality females. Theoretical and empirical studies suggest that sons of high-quality mothers might also be more likely to settle in high-quality habitats or groups than sons of low-quality mothers [38] , [39] because their better nutritional state allows them to invest more resources in terms of time and energy in assessing potential dispersal destinations. In this study, we tested whether maternal quality affects fitness and the reproductive value of sons in spotted hyaenas. We used 14 years of detailed demographic and life history data and microsatellite profiling of all members of the eight resident clans on the floor of the Ngorongoro Crater (the 'Crater') in Tanzania, a habitat in which anthropogenic effects are limited and processes of natural selection are still intact. We tested whether maternal social status influenced the growth rate of sons during the nursing period, their survival to immigration, their likelihood of immigration into the best clan in terms of fitness prospects, their age at first reproduction and their tenure after immigration. Because male quality may be important to females while choosing a mate [40] we investigated whether females preferred sons of high-ranking mothers. We also investigated whether maternal social status influenced the reproductive performance of sons by assessing the realized annual fitness of immigrant males. Finally, because offspring performance might be influenced by both maternal environmental effects and direct paternal genetic effects, we compared the longevity of offspring sired by males with different maternal social status. We demonstrate that high-born sons grew at higher rates than lower-born sons and gained fitness benefits during adulthood from their privileged upbringing. Our results show that the maternal environment can have profound life history consequences for dispersing males, even in mammal societies in which male fitness depends on how well male behaviour conforms to female mate-choice preferences rather than male size or fighting ability. Growth rates of sons Maternal social status strongly and positively influenced growth rate of sons to the age of 6 months (general linear model, F 2,35 =10.22, P =0.0003, r 2 =0.76), which is a period when offspring entirely depend on milk supplied by their mother [41] . Sons of high-ranking females ( N =25) grew at a rate of 85.2 ± 2.6 g per day (adjusted mean from the general linear model), significantly faster than sons of mid-ranking (71.4 ± 3.5 g per day, N =16, P =0.0033) or low-ranking females (66.7 ± 3.6 g per day, N =11, P =0.0007; Fig. 2 ). The growth rate of sons also depended on (i) the cohort to which the offspring belonged (F 11,35 =5.82, P <0.0001), (ii) litter size and within-litter dominance relationship (F 2,35 =14.51, P <0.0001), in that singletons ( N =8) had higher growth rates than did dominant ( N =19, P =0.011) or subordinate ( N =25, P <0.0001) siblings from twin litters, and dominant twin litter siblings had higher growth rates than did subordinate twin litter siblings ( P =0.018) and (iii) maternal experience (F 1,35 =5.72, P =0.022), in that sons of experienced females ( N =29) grew significantly faster than did sons of inexperienced females ( N =23). 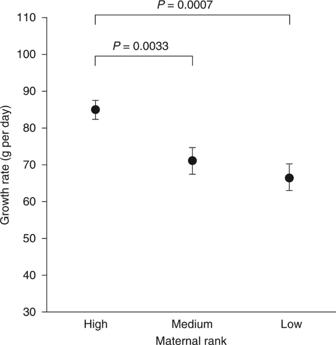Figure 2: The growth rate until the age of 6 months of sons of mothers of different social status. Growth rates are adjusted means±standard errors, as determined by using a general linear model that considered the following variables: maternal rank, cohort, litter size and within-litter dominance relationship, and maternal experience. Figure 2: The growth rate until the age of 6 months of sons of mothers of different social status. Growth rates are adjusted means±standard errors, as determined by using a general linear model that considered the following variables: maternal rank, cohort, litter size and within-litter dominance relationship, and maternal experience. Full size image Immigration age and survival to immigration There was no evidence that maternal social status influenced the age at which males immigrated into a clan (general linear model, N =114 males, F 2,97 =0.012, P =0.99, r 2 =0.23), after the influence of the identity of the natal clan (F 7,97 =2.42, P =0.025) and the identity of the clan into which males immigrated (F 7,97 =2.14, P =0.046) were controlled for. Sons of high-ranking females ( N =51) immigrated at 3.56 ± 0.13 years of age, sons of mid-ranking females ( N =39) at 3.58 ± 0.13 years of age and sons of low-ranking females ( N =24) at 3.55 ± 0.17 years of age. There was also no evidence that maternal social status influenced the survival of sons to the age at adulthood ( Z =1.72, P =0.086) after the influence of litter size and within-litter dominance relationship (dominant surviving better than subordinate: Z =2.05, P =0.04; singleton versus subordinate: Z =1.56, P =0.12) were controlled for (binary logistic regression model, N =394 sons, χ 2 =8.02, degrees of freedom (d.f. )=3, P =0.046), or the survival of sons to the mean age at immigration ( Z =1.81, P =0.070; binary logistic regression model, N =328, χ 2 =3.31, d.f.=1, P =0.069) or their overall longevity ( Z =−0.98, P =0.33) after the influence of the cohort in which they grew up in ( Z =−1.72, P =0.086) was controlled for (survival analysis, Cox proportional hazards model, N =394, G =4.21, d.f.=2, P =0.12). Pattern of immigration We have previously shown that males that immigrate into clans with the highest number of young females (between 1 and 5 years of age) have a substantially higher long-term reproductive success than do other males [27] because young females prefer recent immigrants as sires of their offspring [27] , [29] . To test whether maternal quality influenced the likelihood of dispersing sons to join the clan that offered the highest long-term benefit, we ranked the eight clans according to the number of young females that each clan contained, tallied the number of immigrations into each clan and compared this with the expected number of immigrations on the basis of a random distribution. The observed pattern of immigration of sons of high-ranking mothers ( N =51) significantly deviated from random expectation ( χ 2 =18.61, d.f.=7, P =0.0095), with high-born sons immigrating more often than expected into clans with the highest number of young females ( χ 2 =17.22, d.f.=1, P <0.0001; Fig. 3 ). The pattern of immigration of sons of mid-ranking mothers ( N =39) also deviated from random expectation ( χ 2 =26.94, d.f.=1, P <0.001), but none of the clan ranks were significantly overrepresented. The pattern of immigration of sons of low-ranking mothers ( N =24) did not deviate from random expectation ( χ 2 =9.76, d.f.=7, P =0.20). 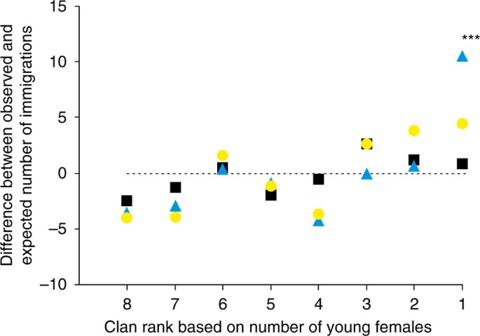Figure 3: The pattern of immigration of sons of mothers of different social status. Clans were ranked by the number of young female clan members on each date of immigration; in each case, the clan with the highest number of young females had rank 1 and the clan with the lowest number of young females had rank 8. Sons of mothers of high (blue triangles), medium (yellow circles) and low (black squares) social status are shown ***P<0.0001. Figure 3: The pattern of immigration of sons of mothers of different social status. Clans were ranked by the number of young female clan members on each date of immigration; in each case, the clan with the highest number of young females had rank 1 and the clan with the lowest number of young females had rank 8. Sons of mothers of high (blue triangles), medium (yellow circles) and low (black squares) social status are shown *** P <0.0001. Full size image Excursions to natal territory After immigration, sons of high-ranking females were more likely to undertake brief feeding excursions to their natal clan territory to benefit from their high natal social status while competing for food with natal clan members than were sons of low-ranking females: (i) the median proportion of short-term excursions to the natal clan territory out of all extraterritorial excursions of high-born sons ( N =36) was higher than that of low-born sons ( N =18; Mann–Whitney U- test, U =205.5, P =0.029) and (ii) the proportion of males that returned to their natal clan territory and maintained their natal rank when feeding there was higher for sons of high-ranking females ( N =22 of 34) than for sons of low-ranking females ( N =5 of 16; χ 2 =4.90, d.f.=1, P =0.027). Males maintained their natal social status in interactions with members of their natal clan in their natal territory for a period of up to 1.6 years (mean=0.7±0.09 years, N =31 males) after their immigration into a clan. Age at first reproduction Maternal social status influenced the age at first reproduction of the 48 immigrant males that sired at least one offspring during this study (general linear model, F 2,34 =8.28, P =0.0011, r 2 =0.52), after the influence of the number of young females present in the new clan at immigration (F 1,35 =5.06, P =0.031), the identity of the new clan (F 7,35 =2.36, P =0.044) and whether males grew up as singletons or as the dominant or subordinate member of a twin litter (F 2,35 =2.71, P =0.081) were controlled for. Sons of high-ranking females ( N =19) sired their first offspring at 4.85 ± 0.28 years of age, significantly younger than did sons of mid-ranking females (5.89 ± 0.27 years of age, N= 21, P =0.027) or sons of low-ranking females (6.76 ± 0.42 years of age, N= 8, P =0.0014; Fig. 4 ). 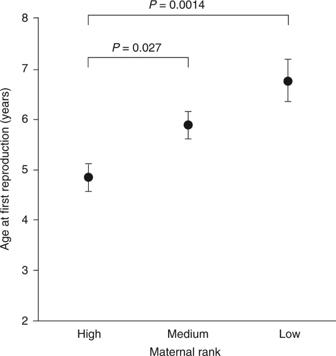Figure 4: The age at first reproduction of sons of mothers of different social status. Ages at first reproduction are adjusted means±standard errors, as determined by using a general linear model that considered the followingvariables: maternal rank, litter size and within-litter dominance relationship, number of young females at immigration, and identity of the new clan. Figure 4: The age at first reproduction of sons of mothers of different social status. Ages at first reproduction are adjusted means±standard errors, as determined by using a general linear model that considered the followingvariables: maternal rank, litter size and within-litter dominance relationship, number of young females at immigration, and identity of the new clan. Full size image Individual contribution to population growth During the study, the size of the hyaena population in the Crater increased on an average by 22.8 ± 6.9 individuals per year, or at a mean annual rate of 8.5 ± 2.4%, from 172 individuals in 1997 to 442 individuals in 2009. The mean annual contribution to population growth by a male that sired one surviving offspring was 0.00156 ± 0.00013 ( N =12 years); it decreased with population size ( y =0.0092−0.0014×ln( x ), with y being the annual contribution to population growth and x being the population size; r 2 =0.67, N =12, P <0.01; Fig. 5 ). A reduction in the age at which surviving offspring are first produced by 1.91 years (the difference in age at first reproduction between sons of high-ranking and low-ranking females) increased the contribution to the population growth of males by 19.1 ± 0.3% (range, 18.0–24.8%). Because sons of high-ranking females sired a mean of 2.37 ± 0.46 offspring during the first 1.91 years after the date of first reproduction, the contribution to population growth of sons of high-ranking females was 45.3% higher than that of sons of low-ranking females. 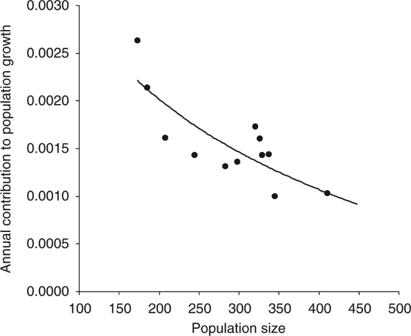Figure 5: The influence of population size on the annual contribution to population growth of males that sired one surviving offspring. The line shows the regression of the annual contribution of males that sired one surviving offspring to population growth by population size,y=0.0092−0.0014×ln(x). Population size was the total number of spotted hyaenas belonging to the eight clans resident on the Crater floor; all spotted hyaenas of these eight clans were individually known. Figure 5: The influence of population size on the annual contribution to population growth of males that sired one surviving offspring. The line shows the regression of the annual contribution of males that sired one surviving offspring to population growth by population size, y =0.0092−0.0014×ln( x ). Population size was the total number of spotted hyaenas belonging to the eight clans resident on the Crater floor; all spotted hyaenas of these eight clans were individually known. Full size image Male tenure and female mate-choice preference Total tenure was similar for sons of high-ranking (mean from the survival analysis=5.7 years, N =51), mid-ranking (mean=6.0 years, N =39) and low-ranking females (mean=5.7 years, N =24; Tarone–Ware χ 2 =1.22, d.f.=2, P =0.54; Fig. 6 ). Maternal social status did not influence the number of cubs per year that males with tenures exceeding 3 years sired during the first 3 years of tenure (general linear model, F 2,41 =1.53, P =0.23, r 2 =0.22) after the positive effect of the number of young females present in the new clan at immigration (F 1,41 =5.65, P =0.022) was controlled for, suggesting a lack of strong female preference for high-born sons. Sons of high-ranking females ( N =15) sired 0.75 ± 0.22 cubs per year (adjusted mean from the general linear model), sons of mid-ranking females ( N =18) sired 0.60 ± 0.20 cubs per year and sons of low-ranking females ( N =12) sired 0.33 ± 0.24 cubs per year during the first 3 years of tenure. 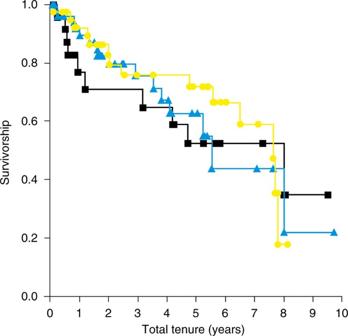Figure 6: Survivorship of adult sons of mothers of different social status during their total tenure as immigrant male. Survivorship is the proportion of males with a total tenure longer than a given tenure. Data include complete tenures as exact values and tenures of individuals still alive at the end of the study as right-censored values. The survivorship curves end in horizontal lines because the males with the longest tenures were still alive at the end of the study. Sons of mothers of high (blue triangles), medium (yellow circles) and low (black squares) social status are shown. Figure 6: Survivorship of adult sons of mothers of different social status during their total tenure as immigrant male. Survivorship is the proportion of males with a total tenure longer than a given tenure. Data include complete tenures as exact values and tenures of individuals still alive at the end of the study as right-censored values. The survivorship curves end in horizontal lines because the males with the longest tenures were still alive at the end of the study. Sons of mothers of high (blue triangles), medium (yellow circles) and low (black squares) social status are shown. Full size image Longevity and paternal genetic effects The maternal rank of the father had no significant influence on the longevity of sons ( Z =0.25, P =0.80), after the influence of the social status of their mother ( Z =−1.05, P =0.29) and the identity of the clan ( Z =−1.45, P =0.15) were taken into consideration (survival analysis, Cox proportional hazards model, G =3.75, N =94 sons that were monitored for up to 8.9 years, d.f.=3, P =0.29), suggesting that direct paternal genetic effects are unlikely to influence the performance of sons. This study demonstrates that the quality of the mother influenced whether sons exercised a preference for high-quality clans at immigration and the age at which their sons started to sire offspring. Do these two parameters influence male reproductive value and success? In spotted hyaenas, male access to females and long-term reproductive success strongly depend on female mate-choice preferences [27] , [29] . To select their mates, females apply simple rules based on male tenure that they use to avoid breeding with close relatives [27] , and they prefer males that build long-term, friendly relationships with them [29] . As a result, males preferentially select clans with the highest number of young females, and males that exercise this preference have a significantly higher long-term reproductive success than do other males [27] . Here, we demonstrated that sons of high-ranking females were more likely to immigrate into clans with the highest number of young females than were sons of lower-ranking females, and we confirmed that the reproductive rate of these immigrant males increased with the number of young females present in the new clan. Thus, high maternal status improved the ability of sons to immigrate into high-quality clans and therefore their long-term reproductive success. Previous studies on spotted hyaenas demonstrated that female mate-choice preferences have several other consequences: with total tenure there is an increase in (i) the reproductive rate of males, (ii) the proportion of offspring sired (of the total reproductive output of males) and (iii) the proportion of females with whom males sire offspring [14] , [29] , [33] . Sons of high-ranking and lower-ranking females in the Crater had similar total tenures and thus were equally likely to be available as sires. Determination of whether male long-term reproductive success depends on age at first reproduction requires the measurement of lifetime reproductive success of high-born and lower-born sons and the assessment of a possible female preference for one or the other category of males. Early reproduction increases a male's likelihood to reproduce before dying. It also increases a male's realized contribution to population growth in expanding populations and thereby its reproductive value, because offspring from early reproduction can contribute to population growth earlier [42] , [43] , [44] . During this study, the hyaena population increased at a mean annual rate of 8.5% and therefore the annual contribution to population growth or 'realized fitness' of males decreased significantly over time. Because sons of high-ranking mothers reproduced at a younger age, their realized fitness and reproductive value were substantially higher than those of sons of low-ranking mothers. In other mammals, individuals that begin reproduction early in life have a shorter adult lifespan or tenure than do other individuals, indicating a trade-off between age at first reproduction and adult survival [45] . In spotted hyaenas, early reproduction does not seem to adversely affect tenure in males, because sons of high-ranking females began reproduction at a younger age but had the same total tenure as sons of lower-ranking females. The apparent lack of a trade-off between early reproduction and longevity in high-born sons may be explained by quality differences between high-born and lower-born sons, strong female mate-choice resulting in low levels of physical conflict between competing immigrant males that queue for status or the absence of male care of offspring [28] , [29] . What are the mechanisms by which maternal status influences the clan into which their sons immigrate and the age at which their sons sire their first offspring? In spotted hyaenas, females of high social status have preferential access to resources and pass their status on to their offspring through behavioural support [15] . As a result, their sons grow faster and have preferential access to resources until they disperse, and for an extended period after this when they return to their natal clan to feed. This may allow sons of high-ranking females to invest more resources in terms of time and energy to search for high-quality dispersal destinations than sons of low-ranking females [38] . Better growth and access to resources in the natal clan territory may also permit sons of high-ranking females to invest more time and energy than sons of low-ranking females in building friendly relationships with females of the new clan, a tactic that increases a male's chance of siring offspring with these females [29] . An earlier age at first reproduction could be a consequence of a female mate-choice preference for males in good condition, that is, for sons of high-ranking females [40] . In this study, sons of high-ranking, mid-ranking and low-ranking females sired a similar number of offspring during the first 3 years of their total tenure, after the influence of the number of young females in the new clan was taken into consideration. We therefore currently have no evidence to suggest that females prefer sons of high-ranking females. We also have no evidence for a strong direct paternal genetic effect, as the longevity of sons of high-born fathers was similar to that of sons of lower-born fathers. We conclude that sons of female hyaenas of high quality benefit from a silver spoon effect. This effect was most likely the result of maternal environmental effects linked to high social status that increased maternal input during the long lactation period in this species [14] and provided sons with privileged access to food resources when weaned. Our findings have important implications for theories of life histories and parental investment [46] , [47] as they demonstrate that the maternal environment experienced during development influenced fitness-related phenotypic traits and reproductive value in dispersing male offspring. They also demonstrate that this even applies to a social mammal with minimal sexual dimorphism and in which male fitness is strongly influenced by female mate-choice preferences rather than fighting ability or body size. Furthermore, by demonstrating for the first time in a non-human mammal [38] that maternal social status can influence patterns of immigration, our study enhances our understanding of dispersal and habitat selection, two key ecological and evolutionary processes. Study area and population The floor of the Ngorongoro Crater in northern Tanzania covers 250 km 2 and is inhabited by eight spotted hyaena clans that defend territories of 24 ± 4 km 2 (Höner et al . [25] ). The Crater population is linked to the neighbouring Serengeti population by individual movements and gene flow [48] . Demographic and behavioural data All spotted hyaenas of the eight clans on the Crater floor were individually known and monitored between April 1996 and September 2009. The social status of adult females was based on the outcome of dyadic interactions using submissive responses [25] . To compare social status across clans, females were assigned a standardized rank by distributing ranks evenly between the highest rank (standardized rank +1) and the lowest rank (standardized rank −1), with the median rank scored as zero. Females with standardized ranks within the top, middle and lower thirds of the total range were then classified as high ranking, mid ranking and low ranking, respectively [28] . Maternal social status was determined for the date of birth of offspring. Individuals were sexed using the shape of their phallic glans [49] . The age of cubs was determined on the basis of pelage, body size, locomotory abilities, behavioural development and position, shape and size of ears [23] , [50] , [51] . Individuals <12 months of age were classified as cubs and those aged between 12 and 24 months as yearlings. Individuals were considered adult when they were ≥24 months of age, because 99.5% of female hyaenas in the Crater ( N =182) conceived their first litter only after 24 months of age and males may have viable sperm in their testes by 24 months of age [52] . However, testosterone concentrations in free-ranging spotted hyaena males indicate that in some males sexual maturity may not occur until after males have immigrated into a new clan [53] , that is, when they are ~3.5 years of age (this study). Clan size was the total number of adult females, cubs, yearlings and adult males of a clan, and population size was the total number of all members of the eight Crater clans. Clan and population sizes were determined on 1 January of each study year. The mean size of Crater clans increased from 21.5 ± 5.0 hyaenas in 1997 to 55.3 ± 8.1 hyaenas in 2009. Individuals were considered to have died or disappeared when their dead body was found or when they were not sighted for at least 1 year. Male immigration pattern To test whether maternal quality influenced the likelihood of males to join clans with the highest number of young females, the eight clans (including each male's natal clan) were placed in a linear rank order on each date that a male immigrated into a clan: rank 1 was the clan with the highest, and rank 8 the clan with the lowest number of young females. The number of immigrations into each clan rank was then tallied and this observed pattern of immigration was compared with the expected pattern based on random distribution by calculating Manly's standardized selection ratio B (=Chesson's α ) [54] . The number of young females included females that were between 1 and 5 years of age. From the perspective of each male, young females in non-natal clans were those between 1 and <5 years of age on the date of clan selection, as recent immigrant males rarely have contact with female cubs <12 months of age [55] . Young females in his natal clan were those that were born before the male's birth and <5 years of age at clan selection. Maternal care and offspring growth Females give birth to one or two, very rarely three, offspring per litter [56] . Cubs are raised at a communal den, and for the first 6 months of their life depend entirely on maternal milk [41] . Crater females nurse their offspring for a mean of 12.6 ± 0.6 months (range 7.3–24.3 months, N =35 females). Growth rates of male cubs were determined for the first 6 months using the mean of three weights measured closest to the age of 6 months, subtracting the average birth mass of 1.5 kg [51] , and dividing the result by the mean age (in days) at which the three weights were taken [41] , [57] . The analysis included weights from 52 males from 41 litters from two clans (27 and 25 males, respectively). Mothers were described as inexperienced when raising their first or second litter and experienced if a particular litter was at least their third litter. Reproductive data In the Crater, the majority of adult males disperse to other clans on the Crater floor and only a small proportion of males disperse elsewhere [27] . For this study, analyses were restricted to the 114 males that were born during the study period and that emigrated from the clan in which they were born and immigrated into another Crater clan without having expressed reproductive activity towards females of their natal clan before emigration. Males immigrated into a clan if they showed affiliative behaviour towards, 'shadowed' or 'defended' [29] females of the clan during a period of at least 3 months or if they joined the male social queue of the clan. Date of immigration was the date of first sighting in the new clan's territory. Total tenure was the number of days from the date of immigration until the date of last sighting. The date of conception of a litter was calculated from litter birth dates on the basis of a gestation period of 110 days [52] . Age at first reproduction was the age at which the first offspring was sired by a male based on genetic paternity analysis. To assess the influence of age at first reproduction on male reproductive value, we calculated the annual contribution to population growth for each individual that was alive at the beginning of a year as outlined in Coulson et al . [44] and determined the regression of population size by individual contribution to population growth of males across all years. To assess individual contribution to population growth, the time interval should be a functional unit of the life cycle of the species studied and it should be shorter than the time it would take for a newborn to reach reproductive age [44] . We consider 1 year as the minimum interbirth interval (95% of 377 interbirth intervals of Crater females are longer than 1 year), and, thus, as a functional time unit of the life cycle of spotted hyaenas. The second condition is also fulfilled because the youngest female hyaena that gave birth in the Crater was 2 years of age. Paternity analysis Genetic material for paternity analysis (tissue, hair, the epithelial layer covering faeces) was collected from 824 Crater individuals, including 679 offspring (70.2% of all known births during the study period), and stored in ethanol or dimethyl sulfoxide (DMSO) salt solution [29] . Fluorescent primers were used to amplify nine highly polymorphic (mean=11.2 ± 1.0 alleles, range 7–15 alleles) microsatellite loci [58] . Paternities were assigned using maximum-likelihood methods as implemented in CERVUS 3.0 [59] . All reproductively active natal males (defined as males that showed affiliative behaviour towards, shadowed or defended females of their natal clan during a period of at least 3 months, or that mated or sired cubs with females of their natal clan [27] ) and immigrant males that were clan members when a litter was conceived were considered to be putative fathers [27] . For 630 offspring (92.8% of all sampled offspring), all candidate males were typed; the mean proportion of candidate males that were typed was 0.986. For 648 (95.4%) of the 679 offspring, paternity was determined with 95% confidence. Only three (0.4%) of the 679 offspring were sired by natal males ( N =2) that were not previously observed to express reproductive interest in females of their natal clan. The mean expected heterozygosity was 0.829, total exclusionary power was 0.999 and the error rate was 0.0041 and was set at 1.0%. Statistical analysis All statistical tests were performed using SYSTAT 13.0 (Systat Software). Results are quoted as means ± standard error, and probabilities are for two-tailed tests. For general linear models, binary logistic regression models and survival analyses using Cox proportional hazards models, independent variables or covariates (maternal social status, identity of natal clan, identity of new clan, maternal experience, cohort, litter size and within-litter dominance relationship and number of young females present at immigration) were included in initial runs and excluded from the final model if they had no significant effect on the dependent variable and increased the Akaike Information Criterion. For the general linear model on the reproductive rate during the first 3 years of total tenure, data for the dependent variable were logarithmically transformed to satisfy the requirement of no significant deviation from normal distribution, as judged by the Lilliefors test. To assess differences between categories in general linear models, we applied Tukey's Honestly Significant Difference post hoc tests that control for the family-wise error rate. Total tenures of males were calculated as non-parametric Kaplan–Meier survivorship functions and incorporated tenures of males that were still alive at the end of the study as minimum estimates (that is, as right-censored data); differences in tenures were calculated using the non-parametric log-rank test [60] . Similarly, the longevity of offspring incorporated individuals still alive at the end of the study as minimum estimates. How to cite this article: Höner, O. P. et al . The fitness of dispersing spotted hyaena sons is influenced by maternal social status. Nat. Commun. 1:60 doi: 10.1038/ncomms1059 (2010).